The transcription factor Apontic-like controls diverse colouration pattern in caterpillars Genetic polymorphisms underlie the convergent and divergent evolution of various phenotypes. Diverse colour patterns on caterpillars, which are ecologically important, are good models for understanding the molecular backgrounds of phenotypic diversity. Here we show that a single evolutionarily conserved gene apontic-like ( apt-like ) encoding for a putative transcription factor accounts for the silkworm p locus, which causes at least 15 different larval markings involved in branch-like markings and eye-spot formation. The expression of apt-like and melanin synthesis genes are upregulated in association with pigmented areas of marking mutants Striped ( p S ) and normal (+ p ) but not in the non-marking allele plain ( p ). Functional analyses, ectopic expression, RNAi and TALEN, demonstrate that apt-like causes melanin pigmentation in a cell-autonomous manner. These results suggest that variation in p alleles is caused by the differential expression of the gene apt-like which induces targeted elevation of gene expressions in the melanin synthesis pathway. The highly diverse colour patterns on caterpillars are of great evolutionary interest because of their association with natural selection [1] , [2] , [3] . Similar to the adult wings of butterflies and moths, their larvae, which are often preyed upon by other animals, also show diverse camouflage and warning-colour patterns [4] , [5] . Some lepidopteran species exhibit highly diverse colour patterns not only among closely related species but also among the same species. The mocker swallowtail Papilio dardanus , an iconic example of Batesian mimicry, can develop distinctly different patterns because of at least 10 gene alleles at a single locus, H [6] , [7] . Heliconius species, which are well known examples of Müllerian mimicry, also display phenotypic diversity in their wing colour patterns [8] , [9] . Both the larvae and adults of various moths are usually cryptically coloured and frequently polymorphic [10] , [11] . Detailed analyses of their developmental processes have revealed how polymorphisms could have been acquired during their evolution. Some of the most convincing data for the genetic and evolutionary control of colour patterns were obtained from different species or spontaneous mutants within species of Drosophila and some butterflies [12] , [13] , [14] , [15] , [16] , [17] , [18] , [19] , [20] , [21] , [22] . In those reports, various genetic changes that contributed to phenotypic differences within or between species were identified; however, the phenomena by which a single locus (gene) can produce multiple phenotypic traits are largely unknown [22] . Because genetic polymorphisms underlie the convergent and divergent evolution of colour pattern diversity [23] , identifying the essential gene that controls this phenotypic diversity is of great interest. Among Lepidoptera, the silkworm Bombyx mori is the most suitable for identifying the gene responsible for colour patterns, because there are numerous pigmentation pattern mutants available, particularly for its larval stages [24] , and its genome sequence and a high-density linkage map are available [25] , [26] . Molecular genetic studies have identified the genes responsible for several colour pattern mutants in the silkworm [27] , [28] , [29] . Turner [30] introduced four different mutations of this silkworm, Moricaud ( p M ), Zebra ( Ze ), Multilunar ( L ) and quail ( q ), which are good models for investigating caterpillar mimicry with various patterns. We previously found that the melanin synthesis genes yellow and ebony were responsible for the silkworm colour mutants chocolate ( ch ) and sooty ( so ) loci, respectively [31] . In addition, we recently found that L resulted from the ectopic expression of Wnt1 in the epidermis [32] . These studies demonstrated that silkworm mutants are useful resources for understanding colour pattern formation. Larval colour patterns primarily depend on the nature and distribution of pigments in epidermal cells and the epicuticle. The normal silkworm (denoted by + p ) pattern comprises three types of spots: (i) eye spots on the second thoracic segment, (ii) crescents on the second abdominal segment and (iii) star spots on the fifth abdominal segment ( Fig. 1a,b ; + p ) [33] . These markings are primarily controlled by one allele (+ p ) of the p locus, which was shown to be located at 3.0 cM of Linkage Group 2 by classical chromosomal mapping [24] . 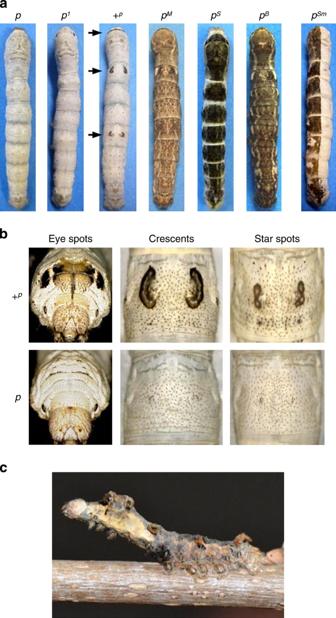Figure 1: Larval marking phenotypes ofBombyx morimutants andB. mandarina. (a) Multiple phenotypes of fifth instar larvae forplocus alleles (except for genetic mosaic strainpSm) of the silkwormB. mori. ThepSmstrain was originally derived from thepSallele by X-ray irradiation44,45. Arrowheads indicate eye spots (upper), crescents (middle) and star spots (bottom). (b) Three kinds of spots reflecting thenormal pattern(+p) and the corresponding region of these markings inplain(p). Note that with thepallele, disc-like structures of normal marking develop but lack black pigmentation. (c) Branch mimicking phenotype of the wild silkwormB. mandarinawith noticeable eye-spot markings on its second thoracic segment. This p locus comprises at least 15 alleles ( Supplementary Table 1 ), which are suitable for studying the molecular background underlying phenotypic polymorphisms. Figure 1: Larval marking phenotypes of Bombyx mori mutants and B. mandarina . ( a ) Multiple phenotypes of fifth instar larvae for p locus alleles (except for genetic mosaic strain p Sm ) of the silkworm B. mori . The p Sm strain was originally derived from the p S allele by X-ray irradiation [44] , [45] . Arrowheads indicate eye spots (upper), crescents (middle) and star spots (bottom). ( b ) Three kinds of spots reflecting the normal pattern (+ p ) and the corresponding region of these markings in plain ( p ). Note that with the p allele, disc-like structures of normal marking develop but lack black pigmentation. ( c ) Branch mimicking phenotype of the wild silkworm B. mandarina with noticeable eye-spot markings on its second thoracic segment. Full size image Among p alleles, plain ( p ) and normal pattern (+ p ) are the most widespread markings among silkworm varieties ( Fig. 1a ). In p larvae, no markings are observed compared with + p larvae ( Fig. 1a,b ; p ). The larval markings of the wild silk moth B. mandarina resemble those of Moricaud ( p M ) of B. mori ; in addition, p M markings of B. mori consist of dark greyish brown lines and dots [33] . Figure 1c shows the branch mimicking of the wild silkworm with noticeable eye-spot markings on the second thoracic segment. These eye spots are also observed on + p larvae ( Fig. 1b ). For Striped ( p S ) larvae, the body surface is solid black, except for the posterior margin of each segment. Several other alleles are known to be located at this locus: Black ( p B ), Ventral striped ( p G ), Whitish striped ( p Sw ), Sable ( p Sa ) and Sable-2 ( p Sa-2 ). The dominance relationship between the major alleles is: p B > p S > p M >+ p > p (ref. 34 ). In this study, we identify apontic-like ( apt-like ) as the gene responsible for these p alleles by positional cloning and functional analyses. We discuss its function and possible roles in pigmentation pattern diversity. Linkage analyses of B. mori p alleles Previously reported linkage analyses mapped 15 p alleles in B. mori to a single chromosomal locus (Linkage Group 2, 3.0 cM) [24] ( Supplementary Table 1 ). 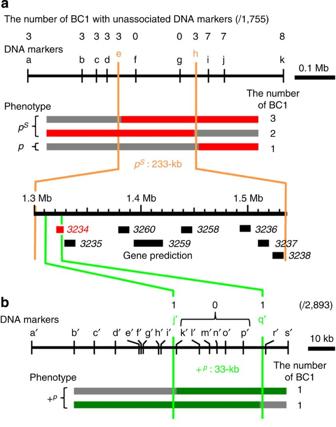Figure 2:plocus positional cloning. (a) Fine mapping of thepSregion and genotypes of informative BC1 selected from 1,755 individuals. Red and grey bars indicate genotypes of heterozygote (pS/p) and homozygote (p/p), respectively. The 233-kb region responsible forpSis denoted by: ‘pS: 233-kb’. The numbers above SNP markers indicate recombination events. Gene prediction was derived from theB. morichina gene model25. (b) Fine mapping of the +pregion and genotypes of informative BC1 selected from 2,893 individuals. Green and grey bars indicate genotypes of heterozygote (+p/p) and homozygote (p/p), respectively. The 33-kb region responsible for +pis denoted by: ‘+p: 33-kb’. The numbers above SNP markers indicate recombination events. To identify the genomic region responsible for these p alleles, we performed low-resolution mapping for 45 back-crossed F1 (BC1) progeny between p and p S individuals using standard single nucleotide polymorphism (SNP) markers (A–F) and fine mapping for 1,710 BC1 progeny using newly designed SNP markers ( Supplementary Table 2 ). Using seven additional SNP markers (a–k in Fig. 2a ), we genotyped 107 individuals among 1,710 BC1 progeny and found that the 233-kb genomic region between markers ‘e’ and ‘h’ of Linkage Group 2 was responsible for the p S phenotype. Figure 2: p locus positional cloning. ( a ) Fine mapping of the p S region and genotypes of informative BC1 selected from 1,755 individuals. Red and grey bars indicate genotypes of heterozygote ( p S / p ) and homozygote ( p / p ), respectively. The 233-kb region responsible for p S is denoted by: ‘ p S : 233-kb’. The numbers above SNP markers indicate recombination events. Gene prediction was derived from the B. mori china gene model [25] . ( b ) Fine mapping of the + p region and genotypes of informative BC1 selected from 2,893 individuals. Green and grey bars indicate genotypes of heterozygote (+ p / p ) and homozygote ( p / p ), respectively. The 33-kb region responsible for + p is denoted by: ‘+ p : 33-kb’. The numbers above SNP markers indicate recombination events. Full size image This region included eight predicted genes ( BGIBMGA003234 , BGIBMGA003235 , BGIBMGA003236 , BGIBMGA003237 , BGIBMGA003238 , BGIBMGA003258 , BGIBMGA003259 and BGIBMGA003260 ) ( Fig. 2a ). Among these genes, cDNA for BGIBMGA003234 was found in four different EST databases for larval tissues with the + p phenotype (CYBERGATE), which suggested that this gene was actively transcribed. In addition, the cDNA for BGIBMGA003234 included sequences for BGIBMGA003235 . This indicated that BGIBMGA003234 and BGIBMGA003235 were categorized as one gene, which was co-transcribed. Thus, we subsequently designated this gene as 3234/5 . Using a similar strategy, we further mapped the genomic region responsible for the p alleles using BC1 progeny of p and + p individuals. We performed fine mapping for 2,893 BC1 progeny and found a 33-kb genomic region responsible for the + p phenotype, which included only the first exon of the gene 3234/5 ( Fig. 2b ). These results indicate that the 3234/5 gene is the most probable candidate for causing the various phenotypes of the p alleles. Structural features of the 3234/5 gene To determine the structural features of the 3234/5 gene, we used rapid amplification of cDNA ends (RACE) and reverse transcription polymerase chain reaction (RT–PCR) for the full-length cDNA structure of the 3234/5 gene from individuals with three different alleles: p , + p and p S . All these genes comprised eight exons, which included a 951-bp open reading frame, encoding 317 amino acids ( Fig. 3a ). When comparing ORFs among the 3234/5 genes for these three alleles, p S 3234/5 included one nucleotide change compared with those of other two alleles, p and + p , which altered Met at the 279-aa site to Thr, while all other amino-acid sequences were the same among these three alleles ( Supplementary Fig. 1 ). 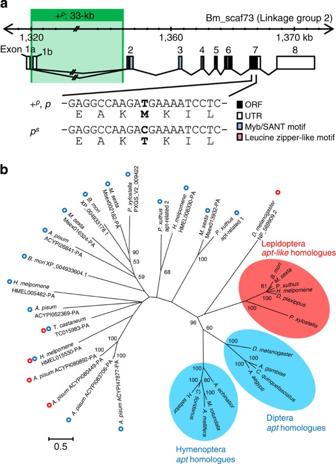Figure 3: Structural features and phylogenetic analysis ofapt-like(3234/5gene). (a) Genomic structure ofapt-likeis shown. Open reading frame (black), untranslated region (white), Myb/SANT motif (blue) and leucine zipper-like motif (red). (b) Unrooted maximum likelihood tree forapt-likeandaptbased on their nucleotide sequences. The numbers at the tree edges represent bootstrap values (1,000 replicates). Only bootstrap value >50% are shown. Branch lengths are scaled to the number of substitutions per site. Red and blue circles indicate Blastp sequence hits (E-value <10−4), obtained with Apt-like or Apt as a query, respectively. These sequences include Myb/SANT motif, but lack a leucine zipper-like motif. Figure 3: Structural features and phylogenetic analysis of apt-like ( 3234/5 gene). ( a ) Genomic structure of apt-like is shown. Open reading frame (black), untranslated region (white), Myb/SANT motif (blue) and leucine zipper-like motif (red). ( b ) Unrooted maximum likelihood tree for apt-like and apt based on their nucleotide sequences. The numbers at the tree edges represent bootstrap values (1,000 replicates). Only bootstrap value >50% are shown. Branch lengths are scaled to the number of substitutions per site. Red and blue circles indicate Blastp sequence hits ( E- value <10 −4 ), obtained with Apt-like or Apt as a query, respectively. These sequences include Myb/SANT motif, but lack a leucine zipper-like motif. Full size image To estimate the function of the gene 3234/5 , we performed a BLAST search using its full-length sequence and found a transcription factor Apontic (Apt), which had a sequence homologous to that of the 3234/5 gene. apt , previously identified in Drosophila melanogaster , is known to be involved in various morphological events, including modifications of the Hox gene, tracheal systems and others [35] , [36] , [37] , [38] , [39] . The Apt protein included a Myb/SANT and a leucine zipper DNA-binding motif, both of which were also retained in the 3234/5 gene ( Fig. 3a , Supplementary Fig. 1b ). Thus, we subsequently designated 3234/5 apt-like . In the lepidopteran species M. sexta , P . xylostella , D. plexippus , H. melpomene and P. xuthus , an orthologous sequence of silkworm apt-like was found ( E -value <10 −23 ). A phylogenetic tree constructed based on the nucleotide sequences for apt , apt-like from several insect species ( E -value <10 −4 ) revealed that all apt-like s in Lepidoptera comprised a monophyletic group, which suggested that this gene was highly conserved among lepidopteran species ( Fig. 3b ). In addition, orthologous sequences of Drosophila apt were observed among dipteran and hymenopteran species ( Fig. 3b ). The phylogenetic tree suggested that apt-likes in Lepidoptera were closely related to apts in Diptera and Hymenoptera (bootstrap value of 96%; 1,000 replications). The apt-like -related sequence CG32813 (NP_569909.2) in D. melanogaster , the apt -related sequence LOC101742283 (XP_004933604.1) and LOC101737608 (XP_004933178.1) in B. mori were also found, although these genes did not encode the leucine zipper-like motif ( Fig. 3b ). We further compared the genomic structures surrounding apt-like in B. mori , D. plexippus and H. melpomene , and found that the gene sets in this region were conserved among these three distantly related species ( Supplementary Fig. 2 ). This suggested that apt-like in Lepidoptera may have evolved from the same ancestral sequence. The accession numbers for apt-like from p S , + p and p strains were registered as AB860412, AB860413 and AB860414, respectively. Pigmentation-associated expression of apt-like To determine the cause of phenotypic differences associated with these three alleles ( p , + p and p S ), we examined the apt-like mRNA expression profiles in the larval epidermis by quantitative RT–PCR. During the fourth instar stage, we prepared cDNA from the larval epidermis of the second abdominal segment, for which pigmentation occurs in phenotypes p S (broad band) and + p (crescent markings) but not in p . Interestingly, apt-like mRNA was highly expressed in the epidermis of p S but not that of p , both at the feeding stage (C2) and moulting stage (E1) before any observable pigmentation ( Fig. 4a ). Furthermore, in the second abdominal segment, apt-like mRNA expression was higher in the epidermis of the + p phenotype compared with that in the epidermis of the p phenotype at the feeding stage but not at the moulting stage ( Fig. 4a ). Notably, apt-like mRNA expression was not induced in the third abdominal segment of + p , which had no pigmentation patterns ( Fig. 4b ). In addition, in the second abdominal segment of + p , apt-like mRNA expression in the crescent marking region was higher compared with that in regions other than those with this marking ( Fig. 4c ). These results clearly show that ectopic expression of apt-like is associated with larval marking pattern formation. 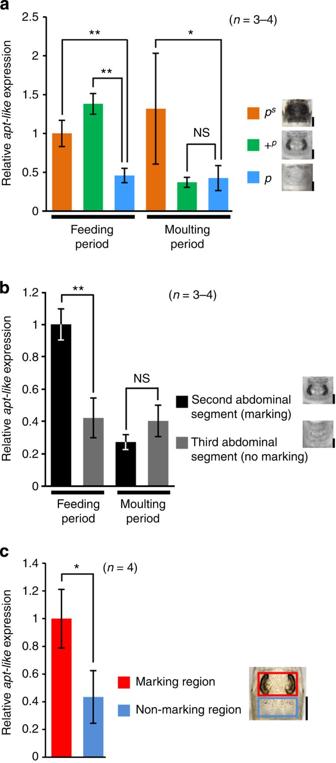Figure 4: Pigmentation associated withapt-likeexpression. (a) Relative expression profiles ofapt-likeamongpS, +pandpalleles as determined by quantitative RT–PCR analysis and plotted as means±s.d. (n=3–4). cDNAs were prepared from the larval epidermis of the second abdominal segment during the fourth instar stage. Feeding period (stage C2) and moulting period (stage E1) were determined based on the spiracle index53. *P<0.05, **P<0.01, Student’st-test. (NS, not significant). Scale bars, 0.2 cm. (b) Relative expression profiles ofapt-likein +palleles as determined by quantitative RT–PCR analysis and plotted as means±s.d. (n=3–4). cDNAs were prepared from the larval epidermis of the second and third abdominal segments during the fourth instar stage. C2 and E1 stages were determined based on the spiracle index. **P<0.01, Student’st-test (NS, not significant). Scale bars, 0.2 cm. (c) Differential expression ofapt-likein the abdominal second segment with the +pallele. Crescent marking region (red box) and non-marking region (blue box) were separately dissected from the same individual and theapt-likemRNA levels were determined by quantitative RT–PCR (n=4). *P<0.05, paired Student’st-test. Scale bar, 0.2 cm. Figure 4: Pigmentation associated with apt-like expression. ( a ) Relative expression profiles of apt-like among p S , + p and p alleles as determined by quantitative RT–PCR analysis and plotted as means±s.d. ( n =3–4). cDNAs were prepared from the larval epidermis of the second abdominal segment during the fourth instar stage. Feeding period (stage C2) and moulting period (stage E1) were determined based on the spiracle index [53] . * P <0.05, ** P <0.01, Student’s t -test. (NS, not significant). Scale bars, 0.2 cm. ( b ) Relative expression profiles of apt-like in + p alleles as determined by quantitative RT–PCR analysis and plotted as means±s.d. ( n =3–4). cDNAs were prepared from the larval epidermis of the second and third abdominal segments during the fourth instar stage. C2 and E1 stages were determined based on the spiracle index. ** P <0.01, Student’s t -test (NS, not significant). Scale bars, 0.2 cm. ( c ) Differential expression of apt-like in the abdominal second segment with the + p allele. Crescent marking region (red box) and non-marking region (blue box) were separately dissected from the same individual and the apt-like mRNA levels were determined by quantitative RT–PCR ( n =4). * P <0.05, paired Student’s t -test. Scale bar, 0.2 cm. Full size image It is known that the pigments caused by the p S and + p alleles consist of melanin [40] . In our previous study, we showed that yellow and ebony mRNA expressions were induced at moulting stages (E1 and E2, respectively), and were more abundant in the p S phenotype compared with that in the + p phenotype [31] . We further compared the mRNA expressions of genes involved in the melanin synthesis pathway and found that Laccase 1 mRNA expression was at similar levels in both phenotypes. However, the mRNA expressions for tyrosine hydroxylase ( TH ), Dopa decarboxylase ( DDC ) and Laccase 2 were induced at higher levels during moulting stages with the p S allele than with the + p allele ( Supplementary Fig. 3 ). These results suggest that apt-like induces downstream melanin synthesis pathway, primarily through yellow and ebony gene expression. Functional analyses of apt-like for larval pigmentation To establish whether our candidate gene apt-like for the p locus caused larval pigmentation, we used a novel technique to ectopically express this gene in vivo [41] . This method enabled the DNA constructs to become integrated into the epidermal genomes using electroporation and resulted in long-term expression of the target gene throughout the larval period. We injected a plasmid that contained both apt-like isolated from the p S strain and enhanced GFP ( EGFP ) genes ( A3-p S apt-like/A3-EGFP ), along with a piggyBac helper plasmid, into the second instar larva of p , which had no pigmentation ( Fig. 5a ). These apt-like -transformed cell lineages could be traced by EGFP fluorescent signals. We used an actin A3 promoter to constitutively express apt-like . 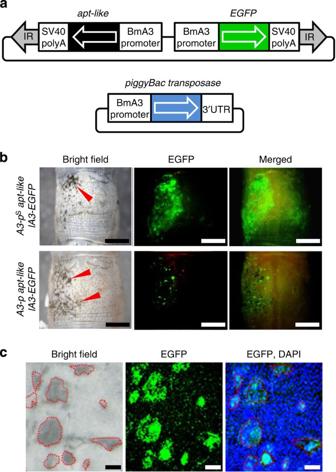Figure 5: Transgenic ectopic expression ofapt-likeinduces black pigmentation on larval cuticles. (a) Schematic representation of thepiggyBacconstruct. Coloured boxes show inserted genes. (b) Transgenic expression in thepallele by electroporation at the fifth instar stage. Upper and lower panels show the results of transgenic expression ofapt-likeisolated frompSandpstrains, respectively. Red arrows indicate ectopic black pigmentation. Scale bars, 0.5 cm. (c) Enlarged areas of ectopic pigmentation (middle panel shows EGFP expression). Epidermal cell nuclei were stained with DAPI (right panel) and pigmented areas (left panel) are enclosed by red lines. Scale bars, 100 μm. Figure 5: Transgenic ectopic expression of apt-like induces black pigmentation on larval cuticles. ( a ) Schematic representation of the piggyBac construct. Coloured boxes show inserted genes. ( b ) Transgenic expression in the p allele by electroporation at the fifth instar stage. Upper and lower panels show the results of transgenic expression of apt-like isolated from p S and p strains, respectively. Red arrows indicate ectopic black pigmentation. Scale bars, 0.5 cm. ( c ) Enlarged areas of ectopic pigmentation (middle panel shows EGFP expression). Epidermal cell nuclei were stained with DAPI (right panel) and pigmented areas (left panel) are enclosed by red lines. Scale bars, 100 μm. Full size image When both plasmids were simultaneously introduced into the left half of a larva, EGFP -positive cells could be observed in the subsequent larval third, fourth and fifth instars ( Fig. 5b ; left sides of fifth instars, EGFP, A3-p S apt-like/A3-EGFP ). Additional melanin pigmentation was observed in the corresponding area of EGFP-positive cells ( Fig. 5b ; bright field, A3-p S apt-like/A3-EGFP ). However, this pigmentation pattern was not observed if negative-control DsRed2 was expressed instead of apt-like ( Supplementary Fig. 4 ). This suggests that pigmentation on the p larval surface is truly induced by transgenic apt-like and not because of unanticipated technical problems. Furthermore, we used quantitative RT–PCR to confirm that apt-like expression introduced in the epidermal cells by the above method was actually upregulated in the EGFP -positive regions ( Supplementary Fig. 5 ). As described above, we noted that p S -Apt-like had one amino-acid change (Met to Thr) at the 279-aa site. Thus, we tested whether this alteration affected the phenotypic differences between p S and p (or + p ) by electroporation-mediated somatic transgenesis [41] . We constructed a plasmid ( A3-p apt-like/A3-EGFP ) that contained apt-like from the p strain rather than apt-like from the p S strain used in the construct described above, which was injected along with the piggyBac helper plasmid into the second instar larva of p and introduced into epidermal cells by electroporation. Similar to the previous results for p S -apt-like , p-apt-like ectopic expression in larval epidermis could also induce pigmentation in the EGFP -positive regions ( Fig. 5b ; bright field, A3-p apt-like/A3-EGFP ). This indicates that the amino-acid changes observed among the three alleles of the p locus are not involved in the protein function of Apt-like, at least with respect to larval pigmentation. In addition, we assessed the detailed pigmentation patterns caused by apt-like ectopic expression using confocal microscopy ( Fig. 5c ). Ectopic pigmentation ( Fig. 5c ; bright field) was generated in the same cells that had EGFP signals ( Fig. 5c ; EGFP), indicated that apt-like regulated the downstream gene activation network during pigmentation processes in a cell-autonomous manner. When short interfering RNA (siRNA) that targeted apt-like was introduced into the left side epidermis of p S or + p at the fourth instar larval stage, melanin pigmentation was blocked for both alleles at the fifth instar stage ( Fig. 6a,b ; right side). However, there was no effect on pigmentation using negative-control siRNA ( Fig. 6a,b ; left side). In addition, inhibition of black pigmentation was observed after introducing apt-like siRNA into p M or p B larvae ( Fig. 6a,b ; right side). These results indicate that a single gene, apt-like , regulates entirely different markings associated with p alleles, and that its expression is necessary for actual pigmentation to occur with all p alleles (at least five) that we tested. 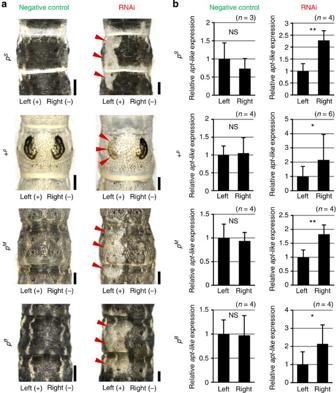Figure 6: Effects ofapt-likesiRNA injection on pigmentation formation for differentpalleles. (a) RNAi effects for thepS, +p,pMandpBalleles. siRNA was introduced by microinjection followed by electroporation. ‘+’ and ‘−’ indicate the electrical current direction during electroporation. For all four differentpalleles, reduced pigmentation was observed only on the ‘+’ sides by siRNA that targetedapt-like(right panel), whereas no effects were observed on pigmentation by negative-control siRNA (left panel). Scale bars, 1 mm. (b) Relativeapt-likeexpression levels in a negative control (left row) and with RNAi (right row) as determined by quantitative RT–PCR analysis and plotted as means±s.d. Numbers of samples are shown at the upper right in each graph. **P<0.01, *P<0.05, paired Student’st-test. (NS, not significant). Figure 6: Effects of apt-like siRNA injection on pigmentation formation for different p alleles. ( a ) RNAi effects for the p S , + p , p M and p B alleles. siRNA was introduced by microinjection followed by electroporation. ‘+’ and ‘−’ indicate the electrical current direction during electroporation. For all four different p alleles, reduced pigmentation was observed only on the ‘+’ sides by siRNA that targeted apt-like (right panel), whereas no effects were observed on pigmentation by negative-control siRNA (left panel). Scale bars, 1 mm. ( b ) Relative apt-like expression levels in a negative control (left row) and with RNAi (right row) as determined by quantitative RT–PCR analysis and plotted as means±s.d. Numbers of samples are shown at the upper right in each graph. ** P <0.01, * P <0.05, paired Student’s t -test. (NS, not significant). Full size image To determine whether apt-like of other lepidopteran species operated on larval pigmentation, we cloned homologous sequences from three swallowtail butterflies, Papilio xuthus , Papilio machaon and Pachiliopta aristrochiae , which are distantly related to B. mori . Sequence alignments revealed that most regions, except for the leucine zipper-like motif, were conserved among apt-like of B. mori and these three swallowtail butterfly species ( Supplementary Fig. 6a ). When these apt-like sequences from butterflies were expressed by in vivo electroporation in the larval epidermis of a p silkworm, melanin pigmentation was observed in regions where it had been introduced ( Supplementary Fig. 6b–d ). These results imply that the putative function of apt-like in melanin pigmentation may be conserved among Lepidoptera. Six predicted genes in p S are not involved in pigmentation Linkage analysis for the p S locus suggested that, in addition to apt-like , six genes ( BGIBMGA003236 , BGIBMGA003237 , BGIBMGA003238 , BGIBMGA003258 , BGIBMGA003259 and BGIBMGA003260 ) were predicted to be within the 233-kb region ( Fig. 2a , Supplementary Fig. 7a ). To determine the possible involvement of these genes in larval pigmentation, we compared the expressions of these genes in the larval epidermis of p S and p strains at the feeding (C2) and moulting (E1) stages ( Supplementary Fig. 7b ). BGIBMGA003237 and BGIBMGA003260 showed higher expressions in the p S epidermis during the feeding stage, whereas the other four genes did not show statistically significant differences in expression between the two alleles at any stage. Of these six genes, BGIBMGA003237 and BGIBMGA003260 were predicted to encode for transcription factors. We knocked down BGIBMGA003237 and BGIBMGA003260 expression by siRNA, which resulted in no effect on pigmentation ( Supplementary Fig. 7c,d ). These results suggest that the six predicted genes are not involved in p S pigmentation and that apt-like is the only promising candidate for p S pigmentation. Isoform expression and functional domains of apt-like We detected several apt-like isoforms in EST databases and by RT–PCR and RACE analyses ( Supplementary Fig. 8a ). To determine the isoform expression for each p allele, we used RT–PCR to amplify the region between exons two and eight of apt-like cDNA prepared from the second abdominal segment of fourth instar larvae. Only a single PCR product was detected in all samples from p , + p and p S larvae; however, its expression appeared to be more abundant in the p S strain ( Supplementary Fig. 8b ). This indicates that the full-length transcript of apt-like is the most abundantly expressed and induced melanin pigmentation in the p S strain. To characterize the functional domain of apt-like exons, we constructed a series of deletion mutants from the C terminus of full-length cDNA ( Supplementary Fig. 9 ). Using electroporation-mediated somatic transgenesis, we co-introduced each plasmid and the piggyBac helper plasmid into second instar larvae and found that exons 3–6 were essential for pigmentation; however, the construct that lacked exon 7 exhibited only weak melanin formation, which suggested that the leucine zipper-like motif was essential for melanin formation in epidermal cells. To confirm this possibility, we tested TALEN-mediated targeted gene knockout in a p S homozygote. To disrupt apt-like , a pair of TALENs that targeted apt-like exon 6, which was just before the leucine zipper-like motif, was designed ( Fig. 7a ; apt-like -TALEN Left and apt-like -TALEN Right). Among TALEN microinjected embryos, two larvae showed white patches among the black stripes of p S ( Fig. 7b ). In these white patched regions, the essential function of apt-like may have been lost in epidermal cells, which could not induce black pigmentation. To determine what kinds of mutations were introduced into the apt-like gene by TALEN, we extracted genomic DNA from two mosaic larvae and amplified the region surrounding the target site by PCR. The sequences of PCR clones showed that two different mutants (Δ6+I11, Δ16) potentially caused the frameshift of apt-like , which broke the coding region of the leucine zipper-like motif ( Fig. 7c ). These results suggest that the leucine zipper-like motif is involved in the essential function of apt-like and support the results described above for knockdown experiments with siRNA. 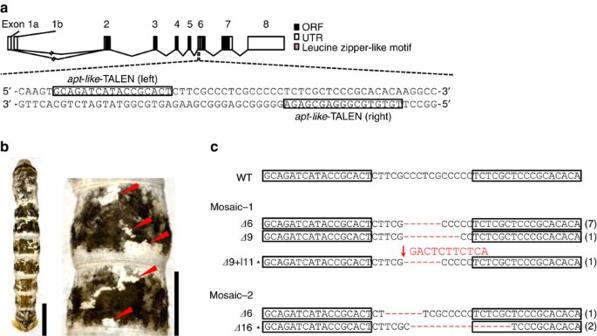Figure 7: Disruption ofapt-likeusing designed transcriptional activator-like effecter nucleases (TALEN). (a) Genomic structure ofapt-likeis shown. Open reading frame (black), untranslated region (white) and leucine zipper-like motif (red). The blue box of exon 6 is expanded to show the gene sequence that includes the 17 bp TALEN binding sites (shown in boxes). (b) Larval mosaic phenotype in G0fifth instar larva ofpStargeted forapt-like. Red arrows indicate remarkable white patches. Photos indicate dorsal overview and magnified view (second and third abdominal segment) in apSmosaic larva, respectively. Scale bars, 1 cm (left photo), 0.5 cm (right photo). (c) Sequences of induced mutations inapt-likefor two mosaic mutants. The wild-type (WT) sequence is shown above the mutant sequences that contain deletions (indicated by red dashes) and insertions (shown by a red arrow and letters). Boxed sequences indicate TALEN binding sites. Asterisks indicate frameshift mutations. The number of clones having identical mutations is indicated to the right of each sequence. Figure 7: Disruption of apt-like using designed transcriptional activator-like effecter nucleases (TALEN). ( a ) Genomic structure of apt-like is shown. Open reading frame (black), untranslated region (white) and leucine zipper-like motif (red). The blue box of exon 6 is expanded to show the gene sequence that includes the 17 bp TALEN binding sites (shown in boxes). ( b ) Larval mosaic phenotype in G 0 fifth instar larva of p S targeted for apt-like . Red arrows indicate remarkable white patches. Photos indicate dorsal overview and magnified view (second and third abdominal segment) in a p S mosaic larva, respectively. Scale bars, 1 cm (left photo), 0.5 cm (right photo). ( c ) Sequences of induced mutations in apt-like for two mosaic mutants. The wild-type (WT) sequence is shown above the mutant sequences that contain deletions (indicated by red dashes) and insertions (shown by a red arrow and letters). Boxed sequences indicate TALEN binding sites. Asterisks indicate frameshift mutations. The number of clones having identical mutations is indicated to the right of each sequence. Full size image Regulatory gene network between apt-like and Wnt1 signalling We previously showed that the ectopic expression of Wnt1 caused melanin pigmentation in the larval epidermis of the + p phenotype [32] . Here we attempted to determine the genetic pathways among apt-like , Wnt1 and Distal-less ( Dll ), using in vivo electroporation as described above. Dll is known to respond directly to morphogen Wnt1 during leg and wing development in Drosophila [42] , [43] . When Wnt1 was ectopically introduced into the larval epidermis of the + p strain, increased expressions of Dll and apt-like were observed and melanin pigmentation occurred ( Fig. 8a,b ; left side). However, Wnt1 ectopic expression in p epidermis could induce the expression of Dll but not that of apt-like or melanin pigmentation ( Fig. 8c,d ; left side). In contrast, apt-like ectopic expression in p larvae caused melanin pigmentation, as shown in Fig. 5 , and induced the expression of Dll but not that of Wnt1 ( Fig. 8e,f ; left side). We further investigated whether Dll expression in the epidermis causes black pigmentation. When siRNA that targeted Dll was introduced into the epidermis of + p and p B as described above, no effects were observed in the both larval pigmentation, which suggested that Dll was not involved in black pigmentation ( Supplementary Fig. 10 ). These results demonstrate that apt-like expression is essential for melanin pigmentation caused by Wnt1. 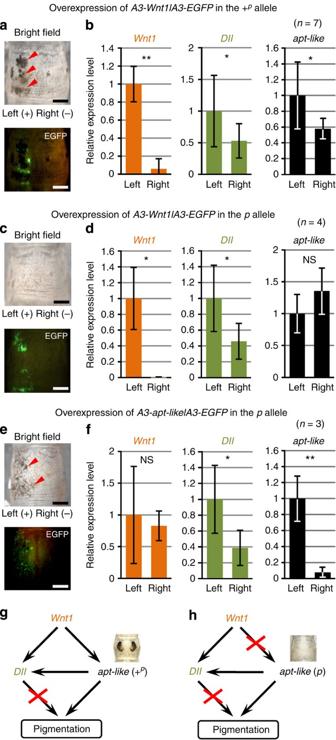Figure 8: Putative gene regulatory network amongWnt1,Dllandapt-like. (a,c)Wnt1transgenic expression by electroporation in the +pallele (a) andpallele (c) for a fifth instar larva, respectively. Red arrows indicate ectopic pigmentation. ‘+’ and ‘−’ indicate the electrical current direction during electroporation. Ectopic pigmentation was observed with the +pallele (a), but not with thepallele (c). Scale bars, 0.5 cm. (b,d) Relative expression levels ofWnt1,Dllandapt-likewith the +pallele (b) andpallele (d), respectively. Error bars indicate s.d. (b,n=7;d,n=4). **P<0.01, *P<0.05, one-tailed paired Student’st-test. (NS, not significant). cDNAs were prepared separately from the left half (includingWnt1-positive cells) and from the right half (withoutWnt1-positive cells as a control) of the epidermis of the abdominal third segment during the fourth instar larval stage (stage C2). (e)apt-liketransgenic expression in thepallele by electroporation for a fifth instar larva. Scale bars, 0.5 cm. (f) Relative expression levels ofWnt1,Dllandapt-likewith thepallele. cDNAs were prepared separately from the left half (includingapt-like-positive cells) and from the right half (withoutapt-like-positive cells as a control) of the epidermis of the abdominal third segment during the fourth instar larval stage (stage C2). Error bars indicate s.d. (n=3). **P<0.01, *P<0.05, one-tailed paired Student’st-test. (NS, not significant). (g,h) Schematic models of the gene regulatory network amongWnt1,Dllandapt-like. (g) With the +pallele,Wnt1has the potential to induce bothDllandapt-likeexpressions.apt-likealso has the potential to induceDllexpression. Black pigmentation is induced byapt-like, but not byDll. (h) With thepallele,apt-likeoriginally has the potential to induce black pigmentation. However, becauseapt-likedoes not have the potential to respond toWnt1, and consequently melanin pigmentation is not induced. Figure 8: Putative gene regulatory network among Wnt1 , Dll and apt-like . ( a , c ) Wnt1 transgenic expression by electroporation in the + p allele ( a ) and p allele ( c ) for a fifth instar larva, respectively. Red arrows indicate ectopic pigmentation. ‘+’ and ‘−’ indicate the electrical current direction during electroporation. Ectopic pigmentation was observed with the + p allele ( a ), but not with the p allele ( c ). Scale bars, 0.5 cm. ( b , d ) Relative expression levels of Wnt1 , Dll and apt-like with the + p allele ( b ) and p allele ( d ), respectively. Error bars indicate s.d. ( b , n =7; d , n =4). ** P <0.01, * P <0.05, one-tailed paired Student’s t -test. (NS, not significant). cDNAs were prepared separately from the left half (including Wnt1 -positive cells) and from the right half (without Wnt1 -positive cells as a control) of the epidermis of the abdominal third segment during the fourth instar larval stage (stage C2). ( e ) apt-like transgenic expression in the p allele by electroporation for a fifth instar larva. Scale bars, 0.5 cm. ( f ) Relative expression levels of Wnt1 , Dll and apt-like with the p allele. cDNAs were prepared separately from the left half (including apt-like -positive cells) and from the right half (without apt-like -positive cells as a control) of the epidermis of the abdominal third segment during the fourth instar larval stage (stage C2). Error bars indicate s.d. ( n =3). ** P <0.01, * P <0.05, one-tailed paired Student’s t -test. (NS, not significant). ( g , h ) Schematic models of the gene regulatory network among Wnt1 , Dll and apt-like . ( g ) With the + p allele, Wnt1 has the potential to induce both Dll and apt-like expressions. apt-like also has the potential to induce Dll expression. Black pigmentation is induced by apt-like , but not by Dll . ( h ) With the p allele, apt-like originally has the potential to induce black pigmentation. However, because apt-like does not have the potential to respond to Wnt1 , and consequently melanin pigmentation is not induced. Full size image Possible models for a gene network among these three genes are shown in Fig. 8g,h . In + p epidermis, Wnt1 induces apt-like and Dll expression, which further induces black pigmentation ( Fig. 8g ). In contrast, in p epidermis, Wnt1 can induce the expression of Dll , but not that of apt-like and black pigmentation ( Fig. 8h ). In both cases, Dll cannot induce melanin pigmentation. In this study, we first focused on differences among three p alleles ( p , + p and p S ) and showed by fine mapping and transgene expression analysis that apt-like was responsible for these alleles. Additional experiments using siRNA knockdown demonstrated that apt-like upregulation was crucial for not only + p and p S but also for p M and p B . These results suggest that apt-like is an essential gene responsible for at least the five alleles that were tested in our study, and its regulatory changes may result in dramatically different larval colour patterns. Based on classical linkage analyses for B. mori , more than 10 pigmentation mutants were mapped exactly at the same p locus ( Supplementary Table 1 ) using thousands of larvae for each analysis. Consequently, the p locus has been shown to be the most remarkable one among hundreds of silkworm mutants [24] . From our results shown here, we anticipate that all of the multiple phenotypes associated with p alleles will be found to be controlled by a single gene, apt-like. Apt has been characterized in Drosophila in four studies, which reported different aspects of the biological functions of this protein. Apt was shown to be a modifier of some Hox gene functions during gnathal development [35] and involved in tracheal cell movement [36] , heart morphology [37] and derepression of oskar translation [38] . Two of these reports indicated that apt may encode for a transcription factor, which may act as a nuclear co-factor for Hox genes [35] , [36] . The Apt protein has glutamine-rich residues and a bZIP motif that includes a potential leucine zipper motif, which implies that this protein homodimerizes or forms a heterodimer with another protein. In addition, Apt includes a putative Myb/SANT DNA-binding domain, which comprises three helix–turn–helix types of alpha-helices. Montell’s group recently discovered that Apt was involved in the expression of an miRNA that regulated JAK/STAT morphogen signalling [39] . Alternatively, Apt was reported to be a cytoplasmic RNA-binding protein involved in the translational control of oskar mRNA [38] ; however, no identifiable RNA-binding motif has been identified for this protein. No reports have indicated that Apt of Drosophila is involved in pigmentation or the melanin synthesis pathway. In our current study, several Apt-like proteins that retained the Myb/SANT motif were found among distantly related lepidopteran species ( Fig. 3b ). Monophyletic apt-like homologues in Lepidoptera were observed at the corresponding chromosomal location of silkworm Linkage Group 2 ( Supplementary Fig. 2 ) and showed highly conserved structures not only in the Myb/SANT motif but also in other coding regions. Injecting siRNA for apt-like into a Bombyx embryo caused its death before hatching, similar to the embryonic lethality of a Drosophila apt mutant [36] . In addition, the EST database showed that silkworm apt-like was expressed in various tissues, including the wing disc, testis, ovary, Malpighian tubule, fat body and trachea. These observations imply that similar to Drosophila Apt, lepidopteran Apt-like has some essential functions for various morphological events other than pigmentation formation on the larval cuticle. The possible function of Apt-like for larval pigmentation was shown to be conserved, at least among Lepidoptera. The important finding of this study is that only one putative transcription factor, Apt-like, is responsible for a single genetic locus, p , which possibly generates phenotypic diversity for pigment patterns. In addition, piggyBac -based somatic transgenesis by electroporation clearly showed that apt-like caused melanin synthesis in a cell-autonomous manner. In addition, TALEN-mediated mosaic analysis showed that somatic apt-like knockout caused white patches among p S markings in a cell-autonomous manner. Our previous reports demonstrated that somatic loss of a chromosomal fragment, including the p S locus, in an epidermal cell-lineage of a genetic mosaic p Sm , mottled striped strain ( Fig. 1 ), produced white patches (variegated pigmentation) among the dorsal black stripes [44] , [45] . The random, impartial loss of this p S chromosomal fragment occurred at any developmental stage, which caused various-sized white spots, even at the single-cell level. These observations supported cell-autonomous functions of apt-like , as shown in this study. In the swallowtail butterfly P. xuthus , expressions of seven melanin-related genes, yellow , tan , ebony , DDC , TH , Laccase 2 and GTPCHI , are strongly correlated with larval eye-spot markings [3] , [31] , [46] , [47] , [48] . Most of these expressions coincide with species-specific cuticle markings of other Papilio species, P. polytes and P. machaon [5] . These observations in butterflies indicate that multiple melanin-related genes located in a separate chromosomal locus act as a module to cause various interspecies and intraspecies pigmentation patterns. In contrast, in Drosophila , alterations in the spatial expression patterns of a small set of melanin synthesis genes, such as yellow , tan and ebony , causes species-specific variations in colour patterns; the expression control of tan and yellow is involved in the divergence of abdominal pigmentation between D. santomea and D. yakuba [49] , [50] . In addition, these few melanin-related genes have been reported to be involved in pigmentation diversity in several Drosophila species [22] , [51] . Although the Apt-like-regulated gene pathway remains unclear, the abundant expression of yellow and ebony is considered to be involved in the dorsal black stripes of the silkworm p S strain [31] . It is noteworthy that the yellow expression coincides with the black regions and is not detected in the white striped region [31] . The weak induction of TH , DDC and Laccase 2 in the p S phenotype after moulting stages ( Supplementary Fig. 3 ) support the above observations and suggest that these melanin synthesis genes act as a module that is co-regulated by Apt-like. We found one amino-acid change among three p alleles; however, this alteration was not involved in the various marking patterns ( Fig. 5b ). apt-like expression was specifically observed in the black stripe regions of p S and the crescent markings of + p ; however, it was severely repressed in p ( Fig. 4a ). In addition, apt-like expression in the pigmentation regions was observed during the feeding stages, which preceded the gene expression of the melanin synthesis module during the moulting phase. These expression profiles of apt-like suggest that the level of gene expression regulates this melanin synthesis module in a region-specific and stage-specific manner. Notably, larval markings should be repeatedly redrawn at each larval moult, which is different from adult pigmentation that occurs only once during metamorphosis. We recently showed that the moulting hormone ecdysteroid possibly regulated larval pigmentation through the function of Wnt1 in lepidopteran spot markings [32] or E75 in eye spots of the swallowtail butterfly [52] . We speculate that in contrast to adult pigmentation, module-type control of gene expression of the melanin synthesis genes is necessary for repeated pigmentation in the larval epidermis. How the region-specific expression of apt-like occurs in the crescent markings of + p is a question that remains to be answered. We recently found a specialized cuticular structure designated ‘bulge’ in the crescent marking area, in which Wnt1 was ectopically expressed and that Wnt1 expression in the larval epidermis had the potential to cause twin spot markings [32] . In this study, using in vivo electroporation, we observed that ectopically expressed Wnt1 induced apt-like expression and melanin pigmentation in + p epidermis but not in p epidermis ( Fig. 8 ). These results suggest that the Wnt1 signalling pathway may be involved in the formation of the crescent markings in + p . It is noteworthy that apt-like ectopic expression could cause melanin pigmentation even in p epidermis, which suggests that the phenotypic differences between p and + p may be generated by their differential responses to the Wnt1 pathway. We speculate that apt-like may be downstream of the Wnt1 pathway in the + p larva ( Fig. 8g ), but not in the p larva ( Fig. 8h ) probably because the cis -regulatory elements of apt-like is mutated and does not respond to the Wnt1 pathway. We compared the sequences in most regions of + p : 33-kb between p and + p strains and observed numerous indels and sequence variations. Thus, some of these variations may be involved in the cis -regulatory changes responsible for binding of Wnt1 signalling factors. In addition, we compared sequences of the + p : 33-kb genomic region among several lepidopteran species, B. mori (surrounding + p : 33-kb as the reference sequence), M. sexta , P. polytes , H. melpomene and D. plexippus by mVISTA, but found no clear homologous regions among them ( Supplementary Fig. 11 ). Detailed, long-range sequence comparisons of each p allele should clarify the regulatory mechanisms for producing phenotypic diversity by only a single novel gene such as apt-like . Silkworm strains The p S mutant strains c05 and f34, + p strains g01 and p20, p M strain u10 and p B strain A10 were from the Institute of Genetic Resources of Kyushu University. The + p strain p50T and p strains N4 and C108 were gifts of Dr T. Shimada (University of Tokyo). The mottled striped strain p Sm 872, which had been induced by X-ray irradiation, was a gift of Dr O. Ninaki (Tokyo University of Agriculture and Technology). Silkworms were reared on mulberry leaves or artificial diets at 25 °C. Staging of fourth instar larvae was based on the spiracle index, which reflects the characteristic sequence of new spiracle formation [53] . Positional cloning of the p S locus For positional cloning of the p S locus, 12 F1 heterozygous males were obtained from a single-pair cross between a p strain N4 male and a p S strain c05 female and each was backcrossed with an N4 female. A total of 1,755 BC1 fifth instar larvae were used for analysis. Genomic DNA was extracted from parent moths, F1 moths and each BC1 of fifth instar larvae using DNAzol solution (Invitrogen). For genetic analysis, 17 SNP–PCR markers were constructed. The primers used for linkage analysis are listed in Supplementary Table 3 . The homozygous (A) or heterozygous (H) state of each BC1 was determined ( Supplementary Table 2 ). Positional cloning of the + p locus For positional cloning of the + p locus, four F1 heterozygous males were obtained from a single-pair cross between a + p strain p50T male and a p strain C108 female and each was backcrossed with a C108 female. A total of 2,893 BC1 of fifth instar larvae were used for the analysis. Genomic DNA was extracted as noted above. For genetic analysis, 39 SNP–PCR markers were constructed. The primers used for linkage analysis are listed in Supplementary Table 4 . The homozygous (A) or heterozygous (H) state of each BC1 was determined ( Supplementary Table 5 ). RT–PCR and RACE Total epidermal RNA was isolated from the silkworm p S mutant strains c05 and f34, + p strains p50T, g01 and p20 and p strain N4 using TRI reagent (Sigma), treated with 0.2 U of DNase I (Takara) at 37 °C for 15 min, purified by phenol–chloroform extraction and then reverse transcribed with a random primer (N6) using a First-Strand cDNA Synthesis Kit (GE Healthcare), according to manufacturers’ protocol. 5′ and 3′ RACE was performed using SMART RACE cDNA Amplification Kit (Clontech), according to the manufacturers’ protocol. PCR products were subcloned into a pGEM-T Easy Vector System (Promega). Nucleotide sequences were determined using an ABI3130xl genetic analyser. Primers used for PCR are listed in Supplementary Table 6 . The gene for ribosomal protein L3 ( rpL3 ) of B. mori was used as an internal control to normalize for equal sample loading. Phylogenetic analysis To determine whether 3234/5 ( apt-like ) orthologues existed in species other than B. mori , we performed phylogenetic analysis using genes included in the Blastp hits ( E- value <10 −4 ) on the NCBI server ( http://www.ncbi.nlm.nih.gov/BLAST/ ), Manduca base ( http://www.agripestbase.org/manduca/ ), Heliconius Genome Project ( http://www.butterflygenome.org/ ), KONAGAbase ( http://dbm.dna.affrc.go.jp/px/ ), BeetleBase ( http://beetlebase.org/ ), AphidBase ( http://www.aphidbase.com/ ) and RNA-seq data for P. xuthus . Apt-like and Apt were used as query for each Blastp search. Codon alignment was generated from a multiple sequence alignment of predicted amino-acid sequences by MUSCLE [54] and PAL2NAL [55] was used to construct nucleotide alignments. The phylogenetic tree was constructed using the maximum likelihood method with the MEGA6 program (GTR+G+I model) [56] . The confidence levels for various phylogenetic lineages were assessed by bootstrap analysis (1,000 replicates). The following sequences were used to create the diagram ( Fig. 3b ): Diptera apt ; D. melanogaster (AAB82746.1), A. gambiae (XP_308214.4), A. aegypti (XP_001652318.1), C. quinquefasciatus (XP_001862892.1). Hymenoptera apt ; A. mellifera (XP_006559097.1), M. rotundata (XP_003708630.1), C. floridanus (EFN69861.1), H. saltator (EFN76284.1), A. echinatior (EGI67737.1). Lepidoptera apt-like ; D. plexippus (EHJ68239.1), M. sexta (Msex004196-PA), H. melpomene (HMEL009522-PA), P. xylostella (PXGS_V2_024627). Quantitative RT–PCR To determine apt-like mRNA expression, we used a Real-Time PCR System with power SYBR green PCR master mix using a StepOne System (Applied Biosystems). Specific primer sets used for target genes are listed in Supplementary Table 6 . The relative expression of a target gene was determined from a standard curve. Expression levels for each sample were determined with no fewer than three biological replicates. We set the normalized apt-like expression level of the far left sample as 1.0 for comparisons with other columns. Statistical comparisons were made by Student’s t -test or paired Student’s t -test. Plasmid construction for piggyBac -based transgene expression We constructed recombinant plasmids from a piggyBac target vector ( pPIGA3GFP::A3DsRed2 ) that contained an EGFP and a DsRed2 marker each driven by a Bm actin A3 promoter. First, the ORF of apt-like was amplified using cDNA from the p S strain c05 and p strain N4 using the PCR primers listed in Supplementary Table 6 . These DNA fragments were used to replace DsRed2 in a piggyBac target vector using an In-Fusion HD Liquid Kit (Clontech). Recombinant plasmids were sequenced using an ABI3130xl genetic analyser to verify nucleotide sequences. Transgene expression piggyBac transposase-based electroporation was performed using a previously described method [41] . The target plasmid that contained the gene of interest ( EGFP marker) and the helper plasmid pHA3PIG , which included piggyBac transposase, were mixed at a final concentration of 1 μg μl −1 each, and 0.5–0.75 μl of this mixture was injected into the haemolymph of second instar larvae of p strain N4 using a glass needle connected to a microinjector (FemtoJet, Eppendorf). Shortly after this injection, electrical stimulation was applied (5 square pulses of 20–25 V, 280 ms width) via two separated small drops of phosphate-buffered saline on the larva, which were used as electrodes to avoid serious damage. siRNA for gene knockdown siRNAs for apt-like were designed that targeted 5′-AACTATAAGAAGAAATGCAAAAT-3′ and 5′-GAGCATACATCCCTTAGACGTCA-3′. siRNAs for BGIBMGA003237 and BGIBMGA003260 were designed to target 5′-TACAATAAAGCAGCCGAAAATGT-3′ or 5′-TTGCATACTCATCTAAACAGACA-3′, respectively. siRNAs for Dll was designed to target 5′-TAGATCATTAGGTTATCCTTTCC-3′ (FASMAC, Japan). Universal negative control siRNA (Nippongene, Tokyo, Japan) was used as a negative control. siRNA (250 μM; 0.5–0.75 μl) was injected from the lateral side of the abdominal fifth segment into haemolymph at the fourth instar larval stage just after moulting. Immediately after injection, phosphate-buffered saline droplets were placed nearby and an appropriate voltage was applied (20 V for the p S , p M and p B alleles; 18 V for the + p allele). Phenotypic effects were observed for fifth instar larvae. To quantify the mRNA levels of target genes by quantitative RT–PCR, the ‘left half’ (into which siRNAs were introduced) and the ‘right half’ of the epidermis were separately dissected from the abdominal third segment ( p S , p M and p B alleles) or the abdominal second segment (+ p allele) of fourth instar larvae (C2 period). TALEN-mediated mosaic analysis Both apt-like -TALEN left and apt-like -TALEN right did not have homologous sequences in the genome. TALEN messenger RNAs were prepared and microinjected into 64 p S embryos using standard protocols [57] . To mutagenise silkworms with this TALEN pair, TALEN left mRNA (200 ng μl −1 ) and TALEN right mRNA (200 ng μl −1 ) were co-injected as a mixture. Among TALEN microinjected embryos, 11 larvae hatched and two larvae became mosaic mutants that had white patches interspersed in a black background. To determine whether mutations had occurred at the specified locus and what types of mutations may have been introduced by TALEN, we extracted genomic DNA from each of these mosaic mutants. The regions surrounding the target sites were amplified by PCR using the appropriate primer sets ( Supplementary Table 6 ), subcloned into a bacterial plasmid and then checked for target sequence modifications. Sixteen clones were examined for each of these mosaic mutants; the frequencies of detected mutant clones were 62.5% (10 per 16 clones) and 18.8% (3 per 16 clones), respectively. Comparative genomics using mVISTA plots The around + p : 33-kb genomic regions of B. mori (chr 2: 1319300-1325400), M . sexta (scaffold00032), H. melpomen e (HE670913_scf7180001249883) and D. plexippus (DPSCF300283) were extracted with KAIKOBASE ( http://sgp.dna.affrc.go.jp/KAIKObase/ ), Manduca Base ( http://agripestbase.org/manduca ), Heliconius Genome Database ( http://www.butterflygenome.org/ ) and MonarchBase ( http://monarchbase.umassmed.edu/ ), respectively. Genomic regions were aligned using the program LAGAN [58] and alignments were visualized using the program mVISTA ( http://genome.lbl.gov/vista/mvista/submit.shtml ). Accession codes : Full-length coding sequences of apt-like from p S , + p and p strains have been deposited in GenBank/EMBL/DDBJ nucleotide core database under the accession codes AB860412, AB860413 and AB860414, respectively. How to cite this article : Yoda, S. et al. The transcription factor Apontic-like controls diverse colouration pattern in caterpillars. Nat. Commun. 5:4936 doi: 10.1038/ncomms5936 (2014).